Role of dopamine D2 receptors in plasticity of stress-induced addictive behaviours Dopaminergic systems are implicated in stress-related behaviour. Here we investigate behavioural responses to chronic stress in dopamine D2 receptor knockout mice and find that anxiety-like behaviours are increased compared with wild-type mice. Repeated stress exposure suppresses cocaine-induced behavioural sensitization, cocaine-seeking and relapse behaviours in dopamine D2 receptor knockout mice. Cocaine challenge after drug withdrawal in cocaine-experienced wild-type or dopamine D2 receptor knockout mice is associated with inhibition of long-term depression in the nucleus accumbens, and chronic stress during withdrawal prevents inhibition after cocaine challenge in cocaine-experienced dopamine D2 receptor knockout mice, but not in wild-type mice. Lentiviral-induced knockdown of dopamine D2 receptors in the nucleus accumbens of wild-type mice does not affect basal locomotor activity, but confers stress-induced inhibition of the expression of cocaine-induced behavioural sensitization. Stressed mice depleted of dopamine D2 receptors do not manifest long-term depression inhibition. Our results suggest that dopamine D2 receptors have roles in regulating synaptic modification triggered by stress and drug addiction. Dopamine regulates emotional and motivational behaviour through the mesolimbic dopaminergic pathway, which projects from the ventral tegmental area to the limbic region, including the nucleus accumbens (NAc), but also to the prefrontal cortex. Dopamine signalling is associated with reward expectation and goal-directed behaviour [1] , [2] . Changes in dopaminergic neurotransmission have been found to modify behavioural responses to various environmental stimuli associated with reward demand. Disturbance of this pathway can result in reduced motivation and anhedonia, which can lead to depression [3] , [4] . Stress is thought to be a key factor in the development of depression, and numerous animal studies have shown that stressful events can induce despair and an altered response to reward, which are characteristics of depression in humans [5] , [6] . Evidence from both human and animal studies suggests that the mesolimbic dopamine system is highly susceptible to stress and is altered by stressful stimuli [6] , [7] , [8] , emphasizing the importance of dopaminergic regulation in the pathophysiology of stress-related behaviour. Chronic or repeated stressful experiences promote adaptive changes in the mesolimbic dopamine system that resemble the chronic actions of several drugs of abuse [9] , [10] , [11] . Indeed, such drugs and stress are thought to induce common neuronal adaptations in the dopaminergic reward system [3] , [12] , [13] . Characterization of the molecular and cellular mechanisms underlying synaptic modification of the mesolimbic dopaminergic system is thus key to an understanding of the interaction between stress and addiction. However, despite the close association of the dopaminergic system with regulation of stress- and addiction-related behaviours, it remains unclear how stress affects the mesolimbic dopaminergic pathway, and especially how long-term stress affects addictive behaviours at the cellular and molecular levels in terms of the synaptic modifications of the dopaminergic system. Dopamine receptors are members of the G protein-coupled receptor family and are classified into D1-like receptors (D1 and D5) and D2-like receptors (D2, D3 and D4). The dopamine D2 receptor (D2R) is highly expressed in the central nervous system and has an important role in the regulation of diverse neural functions by dopamine [14] , [15] , [16] , [17] , [18] , [19] , [20] . It has been shown to act as an autoreceptor in presynaptic regions of the substantia nigra and ventral tegmental area in the midbrain [21] , suggesting that it may have an important role in the central regulation of homeostasis of dopaminergic neurotransmission [18] , [19] , [21] by acting at both the postsynaptic and presynaptic levels. The D2R has also been implicated in various psychiatric and neurological disorders related to addiction, stress, impulsivity and other reward-related behaviours [22] , [23] , [24] , [25] , [26] . We have now investigated the behavioural responses to chronic stress in D2R knockout (D2R −/− ) mice and have found that such mice manifest enhanced anxiety-like and depressive behaviours after such stress compared with wild-type (WT) mice. We also found that repeated stress exposure attenuated cocaine-induced addictive behaviour in association with changes in synaptic plasticity in the NAc in D2R −/− mice. Our results show that D2R has a key role in the interaction between stress and addiction-induced plasticity, and may contribute to relapse after cessation of drug abuse. Anxiety-like behaviours are enhanced in D2R −/− mice WT and D2R −/− mice assigned to ‘stressed’ groups were subjected to restraint stress by immobilization in a restrainer for 30 min, 2 or 6 h in the case of acute stress, and for 2 h daily for 14 days in the case of chronic stress. Control groups of mice were left undisturbed. After stress exposure, the anxiety-like behaviour of the mice was measured with the elevated plus-maze test. Exposure of D2R −/− mice to acute or chronic restraint stress reduced the percentage of entries into and the time spent in the open arms of the maze, as well as the percentage of head dips in the open arms ( Fig. 1a ), whereas the percentage of entries into and the time spent in the closed arms were increased ( Fig. 1c ). The effects of acute or chronic stress on behaviour in this test were significantly greater for the D2R −/− mice than for WT animals ( Fig. 1a–e ). 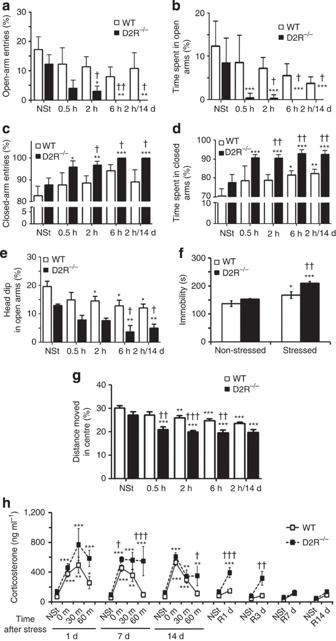Figure 1: Behavioural responses to stress in WT and D2R–/–mice. (a–e) Mice (n≥7 per group) were subjected to the elevated plus-maze test after exposure to restraint stress for 0.5, 2 or 6 h, or for 2 h daily for 14 days. Non-stressed (NSt) animals were examined as a control. The percentage of entries into (a,c) and the time spent in (b,d) the open arms (a,b) or closed arms (c,d), as well as the percentage of head-dipping time in the open arms (e) were determined. (a) Stress effectF4,77=2.7,P=0.036; genotype effectF1,77=12.84,P=0.0006. (b)For NSt versus 2 h/14 day, stress effectF1,30=3.8,P=0.06. (c) Stress effectF4,79=3.29,P=0.0152; genotype effectF1,79=12.11,P=0.0008. (d) Stress effectF4,87=5.11,P=0.001; genotype effectF1,87=23.14,P<0.0001. (e) Stress effectF4,80=5.49,P=0.0006; genotype effectF1,80=36.25,P<0.0001. (f) Immobility time of mice (n=4–10 per group) in the forced swim test after chronic stress (stress effectF1,29=24.28,P<0.0001; genotype effectF1,29=9.35,P<0.0048). (g) Distance travelled by mice (n≥7 per group) in the central zone in the open-field test after acute or chronic restraint stress (stress effectF4,86=14.74,P<0.0001; genotype effectF1,86=53.68,P<0.0001). (h) Plasma concentration of corticosterone in mice (n=6–20 per group) at 0, 30 and 60 min after the end of each stress session on days 1, 7 and 14 of the chronic stress protocol, as well as on days 1, 3, 7 and 14 of recovery (R) after the stress protocol. For 60 min after stress on days 1, 7 and 14: stress effectF1,30>4.29,P<0.05; genotype effectF1,30>10.8,P<0.0026; interactionF1,30>4.29,P<0.05. For day 1 of recovery: stress effectF1,60=9.31,P=0.0034; genotype effectF1,60=11.06,P=0.0015; interactionF1,60=4.01,P=0.0498. For day 3 of recovery: genotype × stress interactionF1,21=1.83,P=0.1906. Two-tailed Student’st-test for (a–d): †P<0.05, ††P<0.01 versus WT mice. One-way analysis of variance (ANOVA)post hoctest fora–d: *P<0.05, **P<0.01, ***P<0.001 versus NSt mice. Two-way ANOVApost hoctest fore–h: *P<0.05, **P<0.01, ***P<0.001 versus NSt mice; †P<0.05, ††P<0.01, †††P<0.001 versus WT mice. All data are means±s.e.m. Figure 1: Behavioural responses to stress in WT and D2R –/– mice. ( a – e ) Mice ( n ≥7 per group) were subjected to the elevated plus-maze test after exposure to restraint stress for 0.5, 2 or 6 h, or for 2 h daily for 14 days. Non-stressed (NSt) animals were examined as a control. The percentage of entries into ( a , c ) and the time spent in ( b , d ) the open arms ( a , b ) or closed arms ( c , d ), as well as the percentage of head-dipping time in the open arms ( e ) were determined. ( a ) Stress effect F 4,77 =2.7, P =0.036; genotype effect F 1,77 =12.84, P =0.0006. ( b) For NSt versus 2 h/14 day, stress effect F 1,30 =3.8, P =0.06. ( c ) Stress effect F 4,79 =3.29, P =0.0152; genotype effect F 1,79 =12.11, P =0.0008. ( d ) Stress effect F 4,87 =5.11, P =0.001; genotype effect F 1,87 =23.14, P <0.0001. ( e ) Stress effect F 4,80 =5.49, P =0.0006; genotype effect F 1,80 =36.25, P <0.0001. ( f ) Immobility time of mice ( n =4–10 per group) in the forced swim test after chronic stress (stress effect F 1,29 =24.28, P <0.0001; genotype effect F 1,29 =9.35, P <0.0048). ( g ) Distance travelled by mice ( n ≥7 per group) in the central zone in the open-field test after acute or chronic restraint stress (stress effect F 4,86 =14.74, P <0.0001; genotype effect F 1,86 =53.68, P <0.0001). ( h ) Plasma concentration of corticosterone in mice ( n =6–20 per group) at 0, 30 and 60 min after the end of each stress session on days 1, 7 and 14 of the chronic stress protocol, as well as on days 1, 3, 7 and 14 of recovery (R) after the stress protocol. For 60 min after stress on days 1, 7 and 14: stress effect F 1,30 >4.29, P <0.05; genotype effect F 1,30 >10.8, P <0.0026; interaction F 1,30 >4.29, P <0.05. For day 1 of recovery: stress effect F 1,60 =9.31, P =0.0034; genotype effect F 1,60 =11.06, P =0.0015; interaction F 1,60 =4.01, P =0.0498. For day 3 of recovery: genotype × stress interaction F 1,21 =1.83, P =0.1906. Two-tailed Student’s t- test for ( a – d ): † P <0.05, †† P <0.01 versus WT mice. One-way analysis of variance (ANOVA) post hoc test for a – d : * P <0.05, ** P <0.01, *** P <0.001 versus NSt mice. Two-way ANOVA post hoc test for e – h : * P <0.05, ** P <0.01, *** P <0.001 versus NSt mice; † P <0.05, †† P <0.01, ††† P <0.001 versus WT mice. All data are means±s.e.m. Full size image WT and D2R −/− mice subjected to chronic stress were also evaluated with the forced swim test. Immobility time in this test is thought to be an indicator of depressive state. The stress-induced increase in immobility time for D2R −/− mice was significantly greater than that for WT mice ( Fig. 1f ). We also analysed locomotor activity in the open-field test, with the level of activity in the centre of the open field being inversely related to anxiety level [27] , [28] , [29] . The distance travelled in the central zone was decreased after acute or chronic stress in WT mice, and this effect was again more pronounced in D2R −/− mice ( Fig. 1g ). We determined the plasma concentration of corticosterone at 0, 30 and 60 min after termination of the stress session on days 1, 7 and 14 of chronic stress, as well as for up to 14 days after the end of the chronic stress protocol in WT and D2R −/− mice. The plasma corticosterone concentration at 0 and 30 min after termination of each stress session was markedly increased in both groups of mice, whereas that at 60 min had returned to near-basal values in WT mice but remained elevated in D2R −/− mice ( Fig. 1h ). The plasma concentration of corticosterone in D2R −/− mice also remained increased for up to 3 days after completion of the stress protocol ( Fig.1h ). Together, these findings suggested that D2R −/− mice manifest increased levels of anxiety-like and depressive behaviours compared with WT animals after exposure to stress. Effect of stress on cocaine-induced sensitization We next explored whether stress might differentially affect other behavioural responses such as addictive behaviours in D2R −/− and WT mice. We first examined behavioural sensitization to repeated administration of cocaine. An initial exposure to psychostimulants, such as cocaine, enhances the locomotor stimulant effect of subsequent drug exposures [30] , [31] . We therefore examined cocaine-induced behavioural sensitization with repeated intraperitoneal (i.p.) injections of cocaine in WT and D2R −/− mice. After habituation to saline injections for 3 days, mice were injected with cocaine (15 mg kg −1 ) on 5 consecutive days, and locomotor responses were recorded for 30 min after each injection ( Fig. 2a ). Both WT and D2R −/− mice showed a marked increase in locomotor activity in response to the repeated cocaine injection ( Fig. 2b ). D2R −/− mice thus manifested cocaine-induced behavioural sensitization similar to that apparent in WT mice, but with the enhancement of the response to the fifth injection of cocaine in D2R −/− mice being greater than that in WT mice as revealed by the ratio of locomotor activity counts on day 5 to those on day 1, despite the lower basal locomotor activity of the mutant animals ( Fig. 2b–e ). The absence of D2R thus did not appear to affect the initiation of behavioural sensitization. We then examined whether repeated stress for 2 weeks might affect such behavioural sensitization ( Fig. 2f ). Chronic stress before the first cocaine exposure did not affect the initiation of cocaine-induced sensitization in either WT or D2R −/− mice ( Fig. 2g–i ). 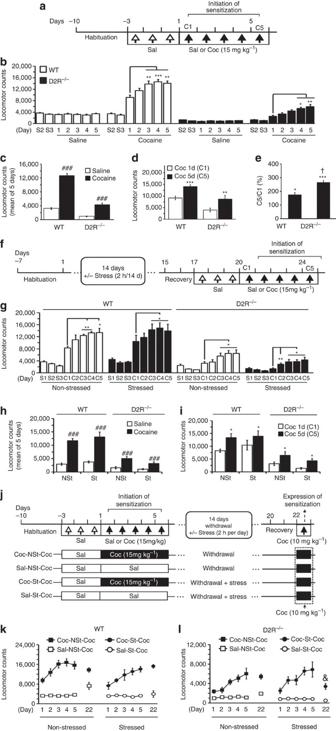Figure 2: Effects of chronic stress before or after repeated cocaine exposure. (a–e) Initiation of sensitization to cocaine (n=16–20 mice per group). (a) Experimental protocol. Sal, saline; Coc, cocaine. (b) Total locomotor counts during 30 min after injection of saline or cocaine (15 mg kg−1, i.p.). (c) Locomotor counts averaged for the five test sessions (cocaine effectF1,65=262.78,P<0.0001). (d) Locomotor activity after the first (day1, C1) and last (day5, C5) injections of cocaine (cocaine day effectF1,54=29.76,P<0.0001; genotype effectF1,54=95.39,P<0.0001). (e) C5/C1 ratio of locomotor counts (cocaine day effectF1,54=27.4,P<0.0001; genotype × cocaine day interactionF1,54=3.9,P=0.0533). (f–i) Effect of chronic stress on initiation of sensitization to cocaine (n=5–8 mice per group). Mice were examined as inathroughewith the addition that they were subjected to restraint stress (St) or not (NSt) for 2 h per day for 14 days before the initiation protocol. (h) For both genotypes, cocaine effectF1,20>40.73,P<0.0001. (i) For both genotypes, cocaine effectF1,16>5.93,P<0.03; cocaine × stress interactionF1,16<0.2,P>0.66. (j–l) Effect of chronic stress on expression of sensitization to cocaine (n=4–11 mice per group). (j) Experimental protocol. (k,l) Locomotor activity of WT (k) and D2R–/–(l) mice during the initiation of behavioural sensitization with five daily injections of cocaine (15 mg kg−1) as well as during the expression of behavioural sensitization induced by challenge with cocaine (10 mg kg−1, i.p.) after drug withdrawal for 14 days with or without stress (each saline versus cocaine pretreatment group two-tailed Student’st-test,P<0.01; expression of sensitization on day 22: (k) stress × cocaine interactionF1,12=4.27,P=0.0610 and (l) cocaine effectF1,16=47.5,P<0.0001). Two-tailed Student’st-test forbandg: *P<0.05, **P<0.01, ***P<0.001. Two-way analysis of variancepost hoctest forc,d e,handi, as well as the expression of sensitization inkandl: *P<0.05, **P<0.01, ***P<0.001 versus the value for C1; ###P<0.001 versus saline control; †P<0.05 versus WT mice; &P<0.05 versus NSt value. All data are means±s.e.m. Figure 2: Effects of chronic stress before or after repeated cocaine exposure. ( a – e ) Initiation of sensitization to cocaine ( n =16–20 mice per group). ( a ) Experimental protocol. Sal, saline; Coc, cocaine. ( b ) Total locomotor counts during 30 min after injection of saline or cocaine (15 mg kg −1 , i.p.). ( c ) Locomotor counts averaged for the five test sessions (cocaine effect F 1,65 =262.78, P <0.0001). ( d ) Locomotor activity after the first (day1, C1) and last (day5, C5) injections of cocaine (cocaine day effect F 1,54 =29.76, P <0.0001; genotype effect F 1,54 =95.39, P <0.0001). ( e ) C5/C1 ratio of locomotor counts (cocaine day effect F 1,54 =27.4, P <0.0001; genotype × cocaine day interaction F 1,54 =3.9, P =0.0533). ( f – i ) Effect of chronic stress on initiation of sensitization to cocaine ( n =5–8 mice per group). Mice were examined as in a through e with the addition that they were subjected to restraint stress (St) or not (NSt) for 2 h per day for 14 days before the initiation protocol. ( h ) For both genotypes, cocaine effect F 1,20 >40.73, P <0.0001. ( i ) For both genotypes, cocaine effect F 1,16 >5.93, P <0.03; cocaine × stress interaction F 1,16 <0.2, P >0.66. ( j – l ) Effect of chronic stress on expression of sensitization to cocaine ( n =4–11 mice per group). ( j ) Experimental protocol. ( k , l ) Locomotor activity of WT ( k ) and D2R –/– ( l ) mice during the initiation of behavioural sensitization with five daily injections of cocaine (15 mg kg −1 ) as well as during the expression of behavioural sensitization induced by challenge with cocaine (10 mg kg −1 , i.p.) after drug withdrawal for 14 days with or without stress (each saline versus cocaine pretreatment group two-tailed Student’s t- test, P <0.01; expression of sensitization on day 22: ( k ) stress × cocaine interaction F 1,12 =4.27, P =0.0610 and ( l ) cocaine effect F 1,16 =47.5, P <0.0001). Two-tailed Student’s t- test for b and g : * P <0.05, ** P <0.01, *** P <0.001. Two-way analysis of variance post hoc test for c , d e , h and i , as well as the expression of sensitization in k and l : * P <0.05, ** P <0.01, *** P <0.001 versus the value for C1; ### P <0.001 versus saline control; † P <0.05 versus WT mice; & P <0.05 versus NSt value. All data are means±s.e.m. Full size image Behavioural sensitization persists after cessation of cocaine administration, with the long-lasting sensitization being known as expression of sensitization [30] , [32] . After induction of behavioural sensitization by repeated injection of cocaine (15 mg kg −1 per day, i.p.) for 5 days, expression of sensitization was evoked by challenge with a lower dose of cocaine (10 mg kg −1 , i.p.) 16 days later (14 days of withdrawal plus 2 days of recovery for stressed groups). Both cocaine- and saline-treated WT or D2R −/− mice were divided into two groups: one group was exposed to restraint stress for 2 h per day during the 14-day withdrawal period, whereas the other group was not subjected to stress during this period ( Fig. 2j ). Repeated stress for 14 days during cocaine withdrawal tended to potentiate the expression of sensitization in WT mice ( Fig. 2k ). For D2R −/− mice, however, although the non-stressed group manifested expression of sensitization, in stressed group the expression of sensitization was significantly attenuated by repeated stress during drug withdrawal ( Fig. 2l , Supplementary Fig. S1 ). Repeated stress during drug withdrawal thus abrogated the expression of cocaine-induced behavioural sensitization in D2R −/− mice (stress effect: F 1,16 =12.86, P =0.0025; P <0.05 versus non-stressed mice; Fig. 2l ). Effect of stress on conditioned place preference To examine the effect of chronic stress on drug-seeking and relapse behaviours, we performed the conditioned place preference (CPP) test with non-stressed and stressed WT and D2R −/− mice. We first tested the effect of chronic stress on the CPP score when the stress session preceded conditioning with cocaine at 15 mg kg −1 ( Fig. 3a ). Both non-stressed and stressed WT and D2R −/− mice showed a similar preference for the drug-paired context ( Fig. 3b ). In a second experiment, mice were subjected to chronic stress between conditioning with cocaine (15 mg kg −1 ) and the CPP test ( Fig. 3c ). Although WT mice showed an increased conditioning score after chronic stress, D2R −/− mice showed a significant decrease in CPP score (genotype × stress interaction: F 1,12 =21.67, P =0.0006; Fig. 3d ). Moreover, non-stressed D2R −/− mice exhibited a higher conditioning score than did non-stressed WT mice. These data suggested that repeated stress enhanced the expression and retrieval of addictive behaviour in WT mice but suppressed such behaviour in D2R −/− mice. 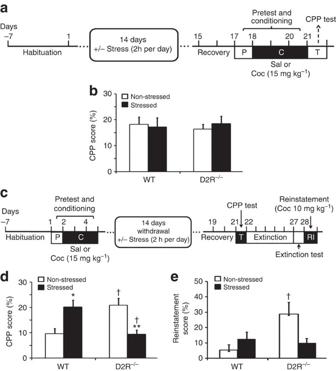Figure 3: Effects of chronic stress on expression and reinstatement of cocaine-induced CPP in WT and D2R–/–mice. (a) Experimental protocol for determination of the effect of chronic stress implemented before cocaine conditioning on the expression of CPP (P, pretest; C, conditioning; T, CPP test). (b) CPP score for the protocol inawas calculated as the percentage of time spent by mice (n=4 per group) in the cocaine-paired compartment during the test session minus the percentage of time spent in the same compartment during the pretest session (genotype effectF1,12=0.01,P=0.9229; stress effectF1,16=0.03,P=0.8547; interactionF1,12=0.31,P=0.5897). (c) Experimental protocol for determination of the effects of chronic stress during withdrawal after cocaine conditioning on cocaine-induced CPP and cocaine-primed reinstatement (RI) as shown indande, respectively. (d) CPP score (n=4 per group, stress effectF1,12=0.0448,P=0.836; genotype × stress interactionF1,12=21.67,P=0.0006). (e) Cocaine-primed RI of CPP (n=3–4 mice per group, genotype × stress interactionF1,10=7.57,P=0.025). The RI score was calculated as the percentage of time spent in the cocaine-paired compartment during the RI session minus the percentage of time spent in the same compartment during the extinction test session. Two-way analysis of variancepost hoctest: *P<0.05, **P<0.01 versus non-stressed (NSt) mice; †P<0.05 versus WT mice. All data are means±s.e.m. Figure 3: Effects of chronic stress on expression and reinstatement of cocaine-induced CPP in WT and D2R –/– mice. ( a ) Experimental protocol for determination of the effect of chronic stress implemented before cocaine conditioning on the expression of CPP (P, pretest; C, conditioning; T, CPP test). ( b ) CPP score for the protocol in a was calculated as the percentage of time spent by mice ( n =4 per group) in the cocaine-paired compartment during the test session minus the percentage of time spent in the same compartment during the pretest session (genotype effect F 1,12 =0.01, P =0.9229; stress effect F 1,16 =0.03, P =0.8547; interaction F 1,12 =0.31, P =0.5897). ( c ) Experimental protocol for determination of the effects of chronic stress during withdrawal after cocaine conditioning on cocaine-induced CPP and cocaine-primed reinstatement (RI) as shown in d and e , respectively. ( d ) CPP score ( n =4 per group, stress effect F 1,12 =0.0448, P =0.836; genotype × stress interaction F 1,12 =21.67, P =0.0006). ( e ) Cocaine-primed RI of CPP ( n =3–4 mice per group, genotype × stress interaction F 1,10 =7.57, P =0.025). The RI score was calculated as the percentage of time spent in the cocaine-paired compartment during the RI session minus the percentage of time spent in the same compartment during the extinction test session. Two-way analysis of variance post hoc test: * P <0.05, ** P <0.01 versus non-stressed (NSt) mice; † P <0.05 versus WT mice. All data are means±s.e.m. Full size image We further examined the effect of stress on CPP by testing cocaine-induced reinstatement. After performance of the CPP test subsequent to 2 weeks of stress, mice were subjected to an extinction session followed by reinstatement with a lower dose (10 mg kg −1 ) of cocaine ( Fig. 3c ). Although the cocaine-induced reinstatement score was tended to be greater for stressed WT mice than for non-stressed WT mice, it was greater for non-stressed D2R −/− mice than for stressed D2R −/− mice (genotype × stress interaction: F 1,10 =7.57, P =0.025; Fig. 3e ). These results thus indicated that repeated stress potentiates cocaine-seeking behaviour and relapse in WT mice, whereas it blunts these addictive behaviours in D2R −/− mice. Altered cocaine-induced plasticity in D2R −/− mice Previous studies have shown that α-amino-3-hydroxy-5-methyl-4-isoxazolepropionic acid (AMPA)-sensitive glutamate receptor (AMPAR) expression on the cell surface, as well as the ratio of AMPARs to N -methyl-D-aspartate (NMDA)-sensitive glutamate receptors (NMDARs) in the NAc of rodents are increased after 10–14 days of withdrawal, following repeated administration of cocaine, and that these changes are reversed, in association with a reduction in the magnitude of NMDAR-dependent long-term depression (LTD), after a cocaine challenge injection [32] , [33] , [34] , [35] , [36] , [37] . To examine the synaptic responses associated with cocaine and stress exposure in WT and D2R −/− mice, we recorded field excitatory postsynaptic potentials from core neurons in the NAc and implemented an NMDA-dependent LTD induction protocol (900 pulses at 1 Hz for 15 min) protocol. Both naive WT and D2R −/− mice showed a similar profile of LTD induction ( Fig. 4a ). This LTD was blocked by treatment with the NMDAR antagonist D -2-amino-5-phosphonovaleric acid ( Supplementary Fig. S2 ), confirming that it was NMDAR-dependent. 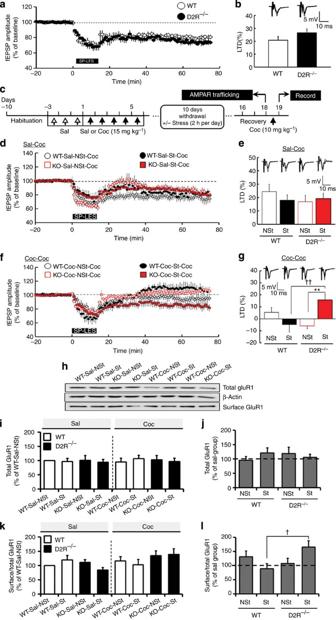Figure 4: Effect of chronic stress on LTD induction in the NAc of cocaine-exposed WT and D2R–/–mice. (a,b) Single-pulse low-frequency stimulation (SP-LFS, 900 pulses at 1 Hz for 15 min) evoked accumbal LTD (a) and bar graph showing the mean percentage LTD at 50–60 min (b) in the NAc core from naive WT and D2R–/–mice (n=6 or 7 mice per group). (c) Experimental protocol for LTD induction (d–g) and AMPAR trafficking (h–l) in the NAc core of WT or D2R–/–mice. (d,f) SP-LFS-induced LTD formation in the indicated groups. Sal, saline; Coc, cocaine; NSt, non-stressed; St, stressed. (e,g) Mean percentage LTD at 50–60 min (n=9 mice per group). (e) Genotype × stress interactionF1,25=0.8924,P=0.3539. (g) Genotype × stress interactionF1,25=11.78,P=0.0021. Representative traces (average of five field potentials) recorded 5 min before (grey) and 1 h after (black) the onset of LTD induction are also shown inb,eandg; dashed line indicates the baseline level. (h) Representative immunoblot analysis of total GluR1 and surface GluR1 in the indicated experimental groups. (i,k) Densitometric quantification of the ratio of total GluR1 to β-actin (i,n=8 mice per group) and the ratio of surface to total GluR1 (k,n=5 or 6 mice per group) in immunoblots. (j,l) Ratio of total GluR1 to β-actin (j) and the ratio of surface to total GluR1 (l) in each cocaine-injected group, normalized by values for the corresponding saline-injected group. Two-way analysis of variancepost hoctest (g,l): **P<0.01, †P<0.05, ††P<0.01 for the indicated comparisons. All data are means±s.e.m. Figure 4: Effect of chronic stress on LTD induction in the NAc of cocaine-exposed WT and D2R –/– mice. ( a , b ) Single-pulse low-frequency stimulation (SP-LFS, 900 pulses at 1 Hz for 15 min) evoked accumbal LTD ( a ) and bar graph showing the mean percentage LTD at 50–60 min ( b ) in the NAc core from naive WT and D2R –/– mice ( n =6 or 7 mice per group). ( c ) Experimental protocol for LTD induction ( d – g ) and AMPAR trafficking ( h – l ) in the NAc core of WT or D2R –/– mice. ( d , f ) SP-LFS-induced LTD formation in the indicated groups. Sal, saline; Coc, cocaine; NSt, non-stressed; St, stressed. ( e , g ) Mean percentage LTD at 50–60 min ( n =9 mice per group). ( e ) Genotype × stress interaction F 1,25 =0.8924, P =0.3539. ( g ) Genotype × stress interaction F 1,25 =11.78, P =0.0021. Representative traces (average of five field potentials) recorded 5 min before (grey) and 1 h after (black) the onset of LTD induction are also shown in b , e and g ; dashed line indicates the baseline level. ( h ) Representative immunoblot analysis of total GluR1 and surface GluR1 in the indicated experimental groups. ( i , k ) Densitometric quantification of the ratio of total GluR1 to β-actin ( i , n =8 mice per group) and the ratio of surface to total GluR1 ( k , n =5 or 6 mice per group) in immunoblots. ( j , l ) Ratio of total GluR1 to β-actin ( j ) and the ratio of surface to total GluR1 ( l ) in each cocaine-injected group, normalized by values for the corresponding saline-injected group. Two-way analysis of variance post hoc test ( g , l ): ** P <0.01, † P <0.05, †† P <0.01 for the indicated comparisons. All data are means±s.e.m. Full size image Both WT and D2R −/− mice were then subjected to an experimental protocol similar to that shown in Fig. 2j , with brain slices being prepared 24 h after the cocaine challenge for measurement of LTD ( Fig. 4c ). Behavioural sensitization was also analysed in these mice, with the results ( Supplementary Fig. S3 ) being similar to those shown in Fig. 2 . For saline-pretreated animals, both non-stressed and stressed groups of WT and D2R −/− mice showed a normal pattern of LTD ( Fig. 4d ). In cocaine-pretreated WT mice, LTD was blunted in both non-stressed and stressed groups ( Fig. 4f ), revealing an inability to elicit LTD in core neurons after cocaine experience; the impairment in LTD tended to be greater for the stressed group than for the non-stressed group, but this difference did not achieve statistical significance. In cocaine-pretreated non-stressed D2R −/− mice, LTD formation was suppressed, showing a pattern similar to that for cocaine-pretreated WT mice ( Fig. 4f ). In contrast, cocaine-pretreated and stressed D2R −/− mice still manifested substantial induction of LTD (genotype × stress interaction: F 1,25 =11.78, P =0.0021; Fig. 4f ), similar to that in saline-pretreated animals, indicative of a markedly altered synaptic response in these mice. We also examined changes in the surface expression of AMPARs, in particular that of the GluR1 subunit [35] , [36] , in mice subjected to the same experimental protocol, but with preparation of brain slices from the NAc core at 12 days after the last of the repeated cocaine injections (that is, without cocaine challenge; Fig. 4c ). Repeated cocaine treatment tended to increase the surface expression of GluR1 in WT mice, and this effect appeared to be reversed by stress. In D2R −/− mice, however, surface expression of GluR1 was not affected by cocaine treatment but tended to be increased by stress during drug withdrawal ( Fig. 4h–l ). Although these differences did not achieve statistical significance, analysis of the ratio of surface to total GluR1 expression in each cocaine-injected group normalized by the corresponding saline-injected group by two-way analysis of variance revealed that the effect of stress differed significantly between WT and D2R −/− mice (genotype × stress interaction: F 1,15 =5.38, P =0.035; Fig. 4l ), indicative of an excitatory synaptic component modification altered by stress in cocaine-exposed D2R −/− mice. Role of D2R in the NAc in stress–drug interaction To assess further the role of D2R in stress–drug interaction, we constructed a lentivirus encoding a short hairpin RNA specific for D2R mRNA (Lenti-shD2R) [25] and delivered it to the NAc core of WT mice to reduce the level of D2R expression. We confirmed that D2R expression was markedly attenuated at both mRNA and protein levels, specifically in the NAc core of mice injected with Lenti-shD2R compared with that in mice injected with a lenti-control virus ( Fig. 5a–c ). One week after such bilateral injection of Lenti-shD2R or Lenti-control into the NAc, we subjected the animals to cocaine-induced behavioural sensitization coupled with chronic stress during the withdrawal period as in Fig. 4c . 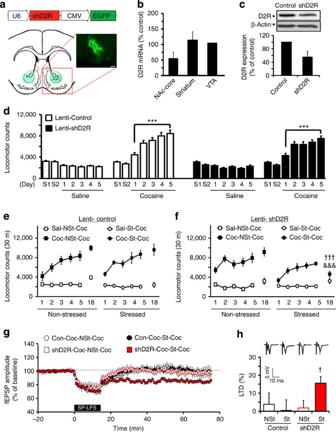Figure 5: Effects of lentivirus-mediated knockdown of D2R in the NAc. (a) Schematic of the lentiviral vector encoding D2R short hairpin RNA (top) and the injection sites (green circles) in the NAc core shown in a coronal diagram of the brain (bottom left). A fluorescence image of enhanced green fluorescent protein (EGFP) expression in the NAc core of a mouse injected with Lenti-shD2R is also shown (bottom right); scale bar, 500 μm. (b) Real-time PCR analysis of D2R mRNA in the NAc core, striatum and ventral tegmental area (VTA). (c) Representative immunoblot analysis of D2R (top) and densitometric quantification of the relative amount of D2R (bottom) in the NAc core of mice injected with Lenti-shDR2 or Lenti-control. (d) Effect of Lenti-shD2R injection into the NAc core on initiation of sensitization to cocaine (n=17–22 mice per group). Total locomotor counts were determined during 30 min after injection of saline or cocaine as inFig. 2a. The first injection of cocaine was administered 1 week after virus injection. (e,f) Effect of Lenti-shD2R injection into the NAc core on expression of sensitization to cocaine. Locomotor activity of mice (n=10-11 per group) injected with Lenti-control (e) or Lenti-shD2R (f) was measured during the initiation and expression of behavioural sensitization to cocaine as inFig. 4c. Expression of sensitization on day 18: (f) stress effectF1,36=9.31,P=0.0043 and stress × cocaine interactionF1,36=11.25,P=0.0019.P<0.01 for each saline- versus cocaine-pretreated group, with the exception of the stressed group injected with Lenti-shD2R (e,f). (g,h) Effect of chronic stress on LTD induction in the NAc of cocaine-exposed mice injected with Lenti-shD2R or Lenti-control into the NAc core (n=7–12 slices per group). Single-pulse low-frequency stimulation-induced LTD formation in the indicated groups (g) and the mean percentage LTD at 50–60 min (h) were determined as inFig. 4c(virus effect × stress interactionF1,31=3.95,P=0.0559). Two-tailed Student’st-test ford, ***P<0.001. Two-way analysis of variancepost hoctest for expression of sensitization ineandf; †††P<0.001 versus mice injected with Lenti-control; &&&P<0.001 versus non-stressed (NSt) mice. All data are means±s.e.m. Figure 5: Effects of lentivirus-mediated knockdown of D2R in the NAc. ( a ) Schematic of the lentiviral vector encoding D2R short hairpin RNA (top) and the injection sites (green circles) in the NAc core shown in a coronal diagram of the brain (bottom left). A fluorescence image of enhanced green fluorescent protein (EGFP) expression in the NAc core of a mouse injected with Lenti-shD2R is also shown (bottom right); scale bar, 500 μm. ( b ) Real-time PCR analysis of D2R mRNA in the NAc core, striatum and ventral tegmental area (VTA). ( c ) Representative immunoblot analysis of D2R (top) and densitometric quantification of the relative amount of D2R (bottom) in the NAc core of mice injected with Lenti-shDR2 or Lenti-control. ( d ) Effect of Lenti-shD2R injection into the NAc core on initiation of sensitization to cocaine ( n =17–22 mice per group). Total locomotor counts were determined during 30 min after injection of saline or cocaine as in Fig. 2a . The first injection of cocaine was administered 1 week after virus injection. ( e , f ) Effect of Lenti-shD2R injection into the NAc core on expression of sensitization to cocaine. Locomotor activity of mice ( n =10-11 per group) injected with Lenti-control ( e ) or Lenti-shD2R ( f ) was measured during the initiation and expression of behavioural sensitization to cocaine as in Fig. 4c . Expression of sensitization on day 18: ( f ) stress effect F 1,36 =9.31, P =0.0043 and stress × cocaine interaction F 1,36 =11.25, P =0.0019. P <0.01 for each saline- versus cocaine-pretreated group, with the exception of the stressed group injected with Lenti-shD2R ( e , f ). ( g , h ) Effect of chronic stress on LTD induction in the NAc of cocaine-exposed mice injected with Lenti-shD2R or Lenti-control into the NAc core ( n =7–12 slices per group). Single-pulse low-frequency stimulation-induced LTD formation in the indicated groups ( g ) and the mean percentage LTD at 50–60 min ( h ) were determined as in Fig. 4c (virus effect × stress interaction F 1,31 =3.95, P =0.0559). Two-tailed Student’s t- test for d , *** P <0.001. Two-way analysis of variance post hoc test for expression of sensitization in e and f ; ††† P <0.001 versus mice injected with Lenti-control; &&& P <0.001 versus non-stressed (NSt) mice. All data are means±s.e.m. Full size image Knockdown of D2R in the NAc core did not affect basal locomotor activity of saline-injected mice or cocaine-induced behavioural sensitization, compared with those observed in mice injected with the control virus ( Fig. 5d ). Such localized depletion of D2R thus did not appear to impair the initiation of behavioural sensitization. In contrast, the expression of sensitization was markedly attenuated by repeated stress during the drug withdrawal period in mice injected with Lenti-shD2R, whereas the non-stressed groups of Lenti-shD2R- or Lenti-control-injected mice manifested significant expression of sensitization ( Fig. 5e ). The alteration of stress-induced drug-seeking behaviour in cocaine-pretreated animals induced by knockdown of D2R in the NAc was thus similar to that apparent in D2R −/− mice ( Fig. 2k ). In a similar set of experiments, we examined the effects of infusion of the D2R antagonist raclopride into the NAc core of WT mice. Such pharmacological blockade of D2R in the NAc showed effects similar to those of D2R knockdown with Lenti-shD2R ( Supplementary Fig. S4 ). To test whether knockdown of D2R in the NAc affects synaptic modification, we prepared brain slices from mice 24 h after the cocaine challenge for measurement of LTD in mice injected with Lenti-shD2R or Lenti-control ( Fig. 5g ). For saline-pretreated animals, both non-stressed and stressed groups of Lenti-control- or Lenti-shD2R-injected mice showed a normal pattern of LTD ( Supplementary Fig. S5 ). For cocaine-pretreated mice injected with Lenti-control, LTD was blunted in both non-stressed and stressed groups ( Fig. 5g ). LTD induction was also suppressed in cocaine-pretreated and non-stressed mice injected with Lenti-shD2R, revealing an inability to elicit LTD in core neurons after cocaine experience. In contrast, cocaine-pretreated and stressed mice injected with Lenti-shD2R still manifested substantial induction of LTD as compared with corresponding mice injected with the control virus ( Fig. 5g ). We have explored the role of D2R in chronic stress responses as well as in the effect of stress on the development and expression of addictive behaviours, providing insight into the interaction between stress and addiction mediated by D2R-dependent modulation of synaptic plasticity. We found that repeated stress promoted anxiety-like and depressive behaviours to a greater extent in D2R −/− mice than in WT mice, and that, in contrast to its effects in WT mice, such stress suppressed the expression of cocaine-induced behavioural sensitization, as well as cocaine-seeking and relapse behaviours in the D2R-mutant animals. As cocaine-induced locomotor activity in non-sensitized (saline-treated) mice was also lower in the stressed mice ( Fig.2l ), one can raise the question whether the suppression of expression of cocaine-induced behavioural sensitization observed in D2R −/− mice may represent an anxiety-induced reduction in activity rather than an interaction between stress and addiction. However, based on our data, this scenario would seem less likely, given that depletion of D2R in the NAc did not affect basal locomotor activity but conferred stress-induced inhibition of the expression of cocaine-induced behavioural sensitization similar to that observed in D2R −/− mice ( Fig.5f ). We therefore propose that chronic stress during drug withdrawal after repeated cocaine exposure results in the recruitment of a D2R-dependent neuroadaptation mechanism that controls the stress-induced increase in cocaine-seeking and relapse behaviours. This stress-induced neuroadaptation interacts with cocaine-induced plasticity in a D2R-dependent manner to reinforce cocaine-seeking and relapse. Such stress-induced neuroadaptation affected the addictive behaviours of cocaine-experienced mice but not those of naive mice, indicating that stress influences cocaine-seeking and relapse rather than the initial acquisition of addictive behaviours. Consistent with this hypothesis, we found that stress-induced synaptic physiology is altered in the NAc of D2R −/− mice. Although cocaine withdrawal after repeated drug exposure attenuated LTD induction in the NAc core after subsequent cocaine challenge in WT mice, and more so in WT mice subjected to repeated stress during the withdrawal period, D2R −/− mice that had been subjected to chronic stress during withdrawal after cocaine exposure manifested a normal pattern of LTD induction in the NAc after cocaine re-exposure. This altered LTD response in the D2R −/− animals was associated with altered surface GluR1 expression in the NAc at the end of the withdrawal period without cocaine re-exposure compared with that in corresponding WT mice. These latter observations might be attributable to a difference in glutamatergic signalling between WT and D2R −/− mice. Glutamatergic synaptic transmission to dopamine neurons is a key site of plasticity [32] , [33] , [34] , [35] , [36] , [37] , [38] , [39] , [40] , and both stress and cocaine directly target NMDARs, which in turn can modulate AMPAR-mediated synaptic transmission [11] . Studies of the effects of acute stress on glutamatergic transmission have shown that such stress enhances synaptic strength by increasing AMPAR trafficking or AMPAR-mediated excitatory transmission in various brain regions, including midbrain dopaminergic neurons, the prefrontal cortex and the NAc shell [41] , [42] , [43] , [44] . However, the effects of chronic stress on glutamatergic signalling are less well understood. Recent studies have indicated that chronic repeated stress reduces AMPAR- and NMDAR-mediated synaptic transmission in the prefrontal cortex, and that AMPAR expression and function in the hippocampus contribute to stress vulnerability [44] , [45] , [46] . Stress-induced secretion of corticosterone results in activation of glucocorticoid receptors, which are important for learning and memory, as well as for synaptic plasticity involving AMPAR trafficking [45] , [46] . We found that D2R −/− mice manifest higher plasma levels of corticosterone after stress, and that these levels return to basal values more slowly compared with WT mice. We therefore cannot rule out the possibility that this impaired corticosterone response results in an altered activation of glucocorticoid receptors in the brain that contributes to the altered stress-induced plasticity associated with regulation of AMPAR trafficking and to the altered drug-craving behaviour in D2R −/− mice. Cocaine-induced alteration of glutamatergic transmission and plasticity involving AMPAR trafficking in the NAc is associated with changes in addiction-related behaviour, notably in cocaine-seeking and relapse [40] , [47] . Long-term withdrawal after repeated cocaine exposure has been shown to enhance excitatory synaptic transmission, in part, through an increase in surface GluR1 expression [33] , [35] , [36] , and this effect is reversed by re-exposure to cocaine [33] , [36] , [40] , [47] . It remains to be determined whether D2R-mediated stress signalling can directly modulate AMPAR trafficking related to GluR1 surface expression. It will also be important to examine how this D2R-dependent stress-induced plasticity interacts only with cocaine-experienced synapses in the transition to relapse. Although it is well accepted that dopaminergic mechanisms mediate cocaine-induced addictive behaviours, the precise contribution of D2R remains to be determined. It has been suggested that the activation of postsynaptic D2Rs on striatopallidal neurons in the NAc facilitates drug-seeking behaviours, with opposite modulation being mediated by D1Rs [48] , [49] . Although D2R −/− mice manifested a general reduction in locomotor activity, they also exhibited cocaine-mediated behavioural sensitization and drug-seeking behaviours at levels similar to or greater than those observed in WT mice, consistent with previous observations [50] , [51] , [52] . Recent studies have shown that ablation or inhibition of striatal D2R-expressing medium spiny neurons enhanced the sensitivity of mice to amphetamine [53] , [54] . The effects of depletion of D2R in the NAc or microinfusion of a D2R antagonist into this brain region in the present study suggest that D2R contributes to stress-induced relapse to cocaine-seeking, without affecting initial drug acquisition or drug-seeking. Our results therefore provide substantial evidence for a distinct role of D2R in drug-craving and relapse in interaction with chronic stress. How altered regulation of D2R signalling affects synaptic plasticity in association with other neurotransmitter systems such as glutamatergic transmission, and how such interactions contribute to other reward-related behaviours such as impulsivity and eating, await further investigation. In conclusion, we have shown that D2R modulates stress-induced plasticity as well as its interaction with drug-evoked plasticity in addiction. Given that stress-induced D2R-dependent signalling appears key to modulation of cocaine-induced metaplasticity, we propose that D2R is an important mediator of stress-induced drug-seeking and relapse. The identification of molecular substrates of stress-induced D2R-dependent signalling in cocaine-induced plasticity may provide novel targets for therapeutic intervention in drug relapse, the primary target for the treatment of addiction disorders. Mice Most experiments were performed with D2R −/− mice (B6;129S2-Drd2tmllow) obtained from the Induced Mutant Resource at the Jackson Laboratory (Bar Harbor, ME), as described previously [18] , [19] , [20] . The D2R −/− mice and WT littermates used in the initial phase of the study originated from the breeding of D2R +/– heterozygotes, as described previously [14] . Mice were maintained in a specific pathogen-free barrier facility under constant conditions of temperature and humidity, and on a 12-h light, 12-h dark schedule. Animal care and handling were performed in accordance with standards approved by the Institutional Animal Care and Use Committee of Korea University. Mice were injected with cocaine hydrochloride (Johnson Mattney, Edinburgh, UK) dissolved in saline (0.9% NaCl). Behavioural analysis Behavioural experiments were performed with male D2R −/− and WT control mice at 11–13 weeks of age, with the exception of those with mice subjected to electrophysiological analysis, which were performed at 21 days of age. For the experiments, age-matched WT and D2R −/− mice were housed individually and allowed to acclimatize to the cage for 1 week. For each manipulation, mice were transferred to the experimental room 60 min before the onset of the experiment, to allow for habituation and to reduce stress (brightness of the experimental room was 70 lux). Each experimental apparatus was cleaned with 70% ethanol between mice to remove odour cues. Mice assigned to stress groups were restrained in a ventilated acrylic restrainer, fitted to allow the animal to breathe but not to move otherwise. For acute stress, mice were immobilized in the restrainer once for 30 min, 2 or 6 h, whereas for chronic stress they were immobilized for 2 h once daily for 14 days. WT and D2R −/− mice were placed in the home cage for restraint stress. Mice assigned to non-stressed groups were untouched in the home cage, whereas their counterparts were subjected to restraint stress. For initiation of sensitization, mice were habituated to saline injections (i.p.) for 3 consecutive days and were then injected with saline or cocaine (15 mg kg −1 , i.p) on 5 consecutive days. Immediately after each injection, mice were tested for horizontal locomotor activity in an open-field chamber for 30 min as described above. For measurement of the effect of chronic stress on the initiation of sensitization ( Fig. 2f–i ), mice were subjected to restraint stress for 2 h daily for 14 days and were then allowed to recover physically for 2 days before saline injection. For measurement of the effect of chronic stress on expression of sensitization ( Fig. 2j–l ), after the last of the 5 consecutive cocaine injections (days 1–5), mice were subjected to restraint stress for 2 h daily for 14 days (10 days for experiments with juvenile mice) and were then allowed to recover from the physical effects of the stress for 2 days. The expression of behavioural sensitization to cocaine was then determined by injection of a challenge dose of the drug (10 mg kg −1 , i.p.). Criteria for sensitization were based on the coefficient of variation (s.d./mean) for the day 5/day 1 locomotor count ratio in the saline group as described previously [35] . A cocaine-injected mouse was considered sensitized if its increase in activity over the course of cocaine treatment (day 5/day 1 locomotor count ratio) exceeded the coefficient of variation for the saline group. For this analysis, the day 5/day 1 locomotor count ratios were calculated based on locomotor activity during the 30-min period after injection. The place preference chamber contained two large compartments that had distinct visual and tactile cues, and which were separated by a manual guillotine door. One compartment consisted of black and white striped walls and a floor of stainless steel rods in a grid pattern. The other compartment had black walls and a floor of stainless steel mesh. The CPP procedure consisted of three phases: pretest, conditioning and test. To measure the effect of chronic stress (restraint stress for 2 h daily for 14 days) on the CPP test, we performed two experiments. In one experiment, chronic stress was applied at the end of the habituation period ( Fig. 3a ); in the other experiment, it was administered at the end of the conditioning period ( Fig. 3c ). Mice were allowed to recover physically from the effect of restraint stress for 2 days before the next manipulation. A pretest was performed to determine the initial chamber preference. Mice were placed between the two compartments with the door open and were free to explore the entire apparatus for 30 min. The time spent in each compartment was recorded with the use of computer software (Med Associates). To avoid effects of zone variation on preference, we performed conditioning with mice that showed the same zone preference in each experiment. Any animal that spent >55% of the total time in either chamber was removed from the study. Conditioning sessions were performed on 3 consecutive days, twice per day (morning and evening). Animals received cocaine (15 mg kg −1 , i.p.) paired with the non-preferred compartment and saline paired with the preferred compartment; alternatively, as a control mice received saline paired alternately with the two sides. The mice were then immediately confined to one of the compartments for 30 min. The procedure for the test session for expression of CPP was similar to that for the pretest. Mice were placed between the two compartments with the door open and then left to choose a compartment for 30 min. Preference for the cocaine-paired or saline-paired chamber was measured by recording the time spent in each. After the CPP test, animals went through extinction training for 5 consecutive days, twice per day (morning and evening; Fig. 3c ). During these sessions, the animals were injected with saline and then immediately confined to the cocaine- and saline-paired compartments as in the conditioning sessions. On the day after the last extinction session, the mice were tested for extinction of CPP by allowing them to freely explore both chambers for 30 min. They were judged to have extinguished CPP if they spent within 55% of the total time in the drug- or saline-paired compartment. [55] Animals that had not extinguished CPP (~15% of mice) were subjected to an additional 1 to 2 days of extinction training until a preference was no longer observed. The day after the extinction test, mice were challenged with cocaine (10 mg kg −1 , i.p.) and then immediately placed in the test apparatus with the door open for determination of the time spent in each compartment over 30 min. A reinstatement score was then calculated as for the CPP score. Electrophysiology The brain was rapidly removed and placed in an ice-cold dissection buffer (5 mM KCl, 1.23 mM NaH 2 PO 4 , 26 mM NaHCO 3 , 10 mM dextrose, 10 mM MgCl 2 , 0.5 mM CaCl 2 and 212.7 mM sucrose, saturated with 95% O 2 and 5% CO 2 , at pH 7.4). The cerebellum and medial aspects of both hemispheres were removed, and the remaining portions of the hemispheres were then glued, midline side up. Parasagittal brain slices (thickness, 400 μm) containing the NAc were prepared with a vibratome (VT1000P; Leica Microsystems, Heppenheim, Germany) and were incubated for at least 1 h at 28 °C in an artificial cerebrospinal fluid (ACSF) containing 124 mM NaCl, 5 mM KCl, 1.23 mM NaH 2 PO 4 , 26 mM NaHCO 3 , 10 mM dextrose, 1.5 mM MgCl 2 and 2.5 mM CaCl 2 at pH 7.4, and saturated with 95% O 2 and 5% CO 2 . The slices were then transferred to a recording chamber, where they were subjected to continuous perifusion with the oxygenated ACSF at a flow rate of 2 ml min −1 . For recording of extracellular field potentials in the NAc, a concentric bipolar stimulating electrode (FHC, Bowdoinham, ME) was placed at the border of the prefrontal cortex and NAc to stimulate afferent cortical fibres, and recordings were made in the rostral-medial dorsal NAc close to the anterior commissure. Picrotoxin (Sigma, St Louis, MO) at 100 μM was added to the ACSF to block the inhibitory effect of γ-aminobutyric acid-mediated neurotransmission in the NAc. Synaptic responses were recorded with ACSF-filled microelectrodes (1–3 MΩ) and were quantified on the basis of the amplitude of field excitatory postsynaptic potentials in the NAc. Recordings were performed with the use of an AM-1,800 microelectrode amplifier (A-M Systems, Sequim, WA), PG 4000A stimulator (Cygnus Technology, Delaware Water Gap, PA) and SIU-90 isolated current source (Cygnus Technology). Baseline responses were collected at 0.07 Hz with a stimulation intensity that yielded a 50–60% maximal response. LTD was induced by single-pulse low-frequency stimulation (900 pulses at 1 Hz for 900 s). Data from slices with stable recordings (<5% change over the baseline period) were included in the analysis. The experimenters were blind to mouse genotype and treatment type. The responses were digitized and analysed with IGOR software (Wavemetrics, Lake Oswego, OR). Statistical analysis Data are presented as means±s.e.m. and were analysed with the two-tailed Student’s t -test, or with one-way or two-way analysis of variance followed by Bonferroni’s post hoc test. A P -value of <0.05 was considered statistically significant. Other methods Additional experimental procedures are provided in Supplementary Methods . How to cite this article: Sim, H. et al . Role of dopamine D2 receptors in plasticity of stress-induced addictive behaviours. Nat. Commun. 4:1579 doi: 10.1038/ncomms2598 (2013).